Hidden dental diversity in the oldest terrestrial apex predatorDimetrodon Paleozoic sphenacodontid synapsids are the oldest known fully terrestrial apex predators. Dimetrodon and other sphenacodontids are the first terrestrial vertebrates to have strong heterodonty, massive skulls and well-developed labio-lingually compressed and recurved teeth with mesial and distal cutting edges (carinae). Here we reveal that the dentition of Dimetrodon and other sphenacodontids is diverse. Tooth morphology includes simple carinae with smooth cutting edges and elaborate enamel features, including the first occurrence of cusps and true denticles (ziphodonty) in the fossil record. A time-calibrated phylogenetic analysis indicates that changes in dental morphology occur in the absence of any significant changes in skull morphology, suggesting that the morphological change is associated with changes in feeding style and trophic interactions in these ecosystems. In addition, the available evidence indicates that ziphodonty evolved for the first time in the largest known species of the genus Dimetrodon and independently from the ziphodont teeth observed in some therapsids. Early Permian (295–270 Ma) sphenacodontid synapsids are of importance as they are the first large-bodied (up to 300 kg) apex predators in the evolutionary history of terrestrial amniotes [1] . For 25 million years, they dominated the first well-established terrestrial vertebrate communities in terms of both relative abundance and number of species [1] , [2] , [3] , [4] , [5] , eventually giving rise to therapsids, the clade that includes mammals [6] . The longest-lived and most geographically widespread sphenacodontid taxon is Dimetrodon , commonly recognized by its elongate neural spines. Early Permian sphenacodontids have a cranial morphology that is ideally suited for carnivory, with tall, strongly constructed snouts, massive skulls and deep jaws. Their strongly heterodont dentition with enlarged premaxillary and anterior maxillary teeth, often with a diastema between them, and with enlarged anterior dentary teeth formed an effective food trap for capturing and restraining prey items. The presence of rows of pterygoid and palatal teeth in the oral cavity and large surface areas for the attachment of jaw adductor muscles (allowing for kinetic-inertial jaw movement) were probably also effective in holding struggling prey [1] , [7] , [8] . Sphenacodontid teeth are teardrop-shaped in labial view, laterally compressed, and possess sharp mesial and distal carinae. It has been suggested previously that the carinae of some Dimetrodon teeth are serrated [9] , [10] , [11] , [12] , [13] , a condition sometimes referred to as ziphodont [14] , [15] , [16] . The original definition of ziphodonty was created through macroscopic examination of denticulate teeth [14] , [17] . Subsequently, ziphodonty has been categorized into several types in thalattosuchian crocodylomorphs based on the external morphology of the denticles when examined with a scanning electron microscope (SEM) [18] . These types include macro- and microziphodonty, which are characterized by true denticles (a serration with a dentine core and an enamel cap), and false-ziphodonty, serrations that are formed by enamel only. However, it is difficult to distinguish true and false-ziphodont teeth without an histological examination of the internal structure of the denticles. Ziphodonty has played an important role in interpretations of feeding behaviour in theropod dinosaurs [11] , [12] , [13] , [19] , [20] , [21] , [22] , marine reptiles [18] , [23] , [24] , crocodylians [25] and extant varanid lizards [16] , but little is known about the role of ziphodonty in sphenacodontids. The apparent occurrence of ziphodonty in the first large-bodied apex predator Dimetrodon has important implications for our understanding of the evolution of feeding behaviour in the initial stages of terrestrial vertebrate evolution. As predator–prey relationships are often tightly linked, with predators and prey exerting evolutionary pressure on each other in an ‘evolutionary arms race’ [7] , [26] , the acquisition of novel feeding systems undoubtedly had a major impact on the initial establishment of modern-day-type terrestrial ecosystems [5] . Here, we analyse the detailed dental anatomy of sphenacodontids, including, Dimetrodon milleri , D. natalis , D. limbatus , D. grandis , Secodontosaurus obtusidens , Sphenacodon ferocior and Ctenospondylus ninevehensis , and describe them within an evolutionary context in order to unravel the hidden complexity of dentition among the oldest known apex predators. The implications for the evolution of feeding strategies in the first terrestrial ecosystems will also be discussed. The results suggest that there is a higher variation in tooth morphology among sphenacodontids than previously thought. The modifications in tooth morphology take place without concomitant changes in skull morphology, as most sphenacodontids have a constrained skull shape. The first occurrence of cusps and ziphodont teeth in sphenacodontids occur independently from those of therapsids, and these changes in tooth morphology may correlate with the appearance of the first well-established terrestrial ecosystems. Morphology and histology of sphenacodontid teeth Heterodonty is universal among sphenacodontids, and tooth size and shape differs between taxa. There are positions for two or three premaxillary teeth in Dimetrodon ( Fig. 1a,b ), Sphenacodon and Ctenospondylus, and five in Secodontosaurus , the most anteromedial of which is the largest. Dimetrodon , Sphenacodon and Ctenospondylus typically have one or two enlarged anterior maxillary teeth and one enlarged anterior dentary tooth that can be up to twice as long as the remaining cheek teeth (for example, MCZ (Museum of Comparative Zoology) 2779, UCMP (University of California Museum of Paleontology) 34196, MCZ 3386, Fig. 1a,b ). Secodontosaurus also has one or two enlarged anterior maxillary teeth, which are not as large as those of Dimetrodon , Sphenacodon and Ctenospondylus , and lacks an enlarged dentary tooth (MCZ 1124). Therefore, heterodonty is less pronounced in Secodontosaurus . 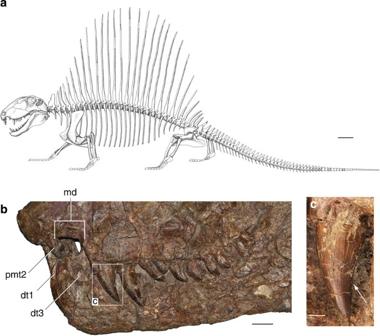Figure 1: Features ofDimetrodon. (a) Reconstruction ofD. limbatus, after Reisz2(reproduced with permission from the author). (b) Snout ofD. limbatus(Museum of Comparative Zoology 2779) in left lateral view. (c) Inset ofbshowing enlarged maxillary tooth with distal cutting edge (white arrow). dt, dentary tooth; md, maxillary diastema; pmt, premaxillary tooth. Scale bars, (a) 10 cm, (b) 2 cm, (c) 1 cm. Figure 1: Features of Dimetrodon . ( a ) Reconstruction of D. limbatus , after Reisz [2] (reproduced with permission from the author). ( b ) Snout of D. limbatus (Museum of Comparative Zoology 2779) in left lateral view. ( c ) Inset of b showing enlarged maxillary tooth with distal cutting edge (white arrow). dt, dentary tooth; md, maxillary diastema; pmt, premaxillary tooth. Scale bars, ( a ) 10 cm, ( b ) 2 cm, ( c ) 1 cm. Full size image The enlarged anterior maxillary teeth of Dimetrodon are nearly conical in cross-section, and frequently have longitudinal ridges in addition to mesial and distal cutting edges ( Fig. 1c ). The remaining cheek teeth of Dimetrodon are tear-drop-shaped in labial view, and intraspecific variation ranges from having blunt, recurved tips and squat bases to being narrower throughout their length with sharper tips. These teeth are more convex labially than lingually, and the tips are recurved distally. The mesial and distal carinae of cf. D. milleri (MCZ 2028) do not possess serrate margins, and are instead formed by smooth, flat, undifferentiated enamel. However, in lingual view, the mesio-distal margin of the tooth bears tiny cusps ( Fig. 2a,b ). The mesial carina curves distally around the base of the lingual side of the tooth, and supports three to four cusps, each 0.1–0.2 mm in width and height. The lingual cusps appear to be above the level of the gum line, which is typically demarcated by the neck of the tooth at the cemento-enamel junction [27] . The teeth of the holotype of D. natalis (AMNH (American Museum of Natural History) 4110) are not well preserved, but one newly prepared area appears to show a smooth distal carina, similar to that of cf. D. milleri . However, the cracked enamel of the tooth may be obscuring any fine detail of the enamel in this specimen, and the presence of lingual cusps cannot be determined. 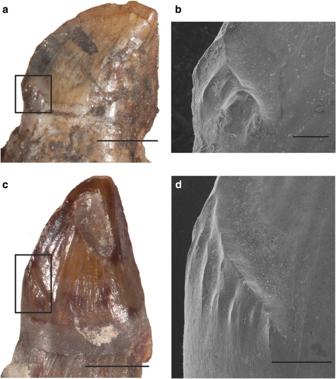Figure 2: cf.D. milleriand cf.D. limbatusteeth. (a) Museum of Comparative Zoology (MCZ) 2028 dentary tooth, lingual view. (b) Scanning electron microscope (SEM) ofashowing cusps on mesial carina. (c) University of Michigan Museum of Paleontology 9778 dentary tooth, lingual view. (d) SEM ofcshowing cusps on mesial carina. Scale bars, (a) 1 mm, (b) 0.2 mm, (c) 2 mm, (d) 0.5 mm. Figure 2: cf. D. milleri and cf. D. limbatus teeth. ( a ) Museum of Comparative Zoology (MCZ) 2028 dentary tooth, lingual view. ( b ) Scanning electron microscope (SEM) of a showing cusps on mesial carina. ( c ) University of Michigan Museum of Paleontology 9778 dentary tooth, lingual view. ( d ) SEM of c showing cusps on mesial carina. Scale bars, ( a ) 1 mm, ( b ) 0.2 mm, ( c ) 2 mm, ( d ) 0.5 mm. Full size image The teeth from the Briar Creek Bonebed, cf. D. limbatus (ROM (Royal Ontario Museum) 64021, UMMP (University of Michigan Museum of Paleontology) 9722), also bear lingual cusps ( Fig. 2c,d ); however, the morphology of the cusps differs from those of cf. D. milleri . The number and size of cusps on each dentary tooth can vary along the tooth row, but on average the lingually curving carina supports five to six cusps. The cusps are taller than wide, each up to 0.5 mm tall and 0.25 mm wide, and are more columnar than those of cf. D. milleri . The carinae in the Briar Creek specimens also differ from those of cf. D. milleri , as they are wavy, and some possess tiny serrations along their margins ( Fig. 3 ). In posterior view, the serrations possess interdentinal sulci ( Fig. 3a ). There are six to seven serrations per mm on the mesial carina, and too many to accurately count on the distal carina, as the keel of each serration is continuous. A thin section through the carina of ROM 64021 shows that the enamel features are built up from a smooth enamel–dentine junction (EDJ), and that the resulting structures are composed of enamel only ( Fig. 3b ). The enamel, although not as clear as when viewed under SEM, resembles synapsid columnar enamel, with continuous, polygonally-shaped columns extending from the EDJ to the outer surface of the tooth [28] , [29] . The teeth of one dentary (StIPB R (Steinman Institute Division of Paleontology, University of Bonn) 598) show a difference in the number of enamel serrations between an unerupted and an erupted tooth of the two enlarged tooth positions in the anterior portion of the dentary ( Fig. 3c–e ). In the unerupted tooth, the serrations are better defined, and are densely packed, with six to seven serrations per mm. In the erupted tooth, the serrations are less well defined and less densely distributed, with only three to four serrations per mm. 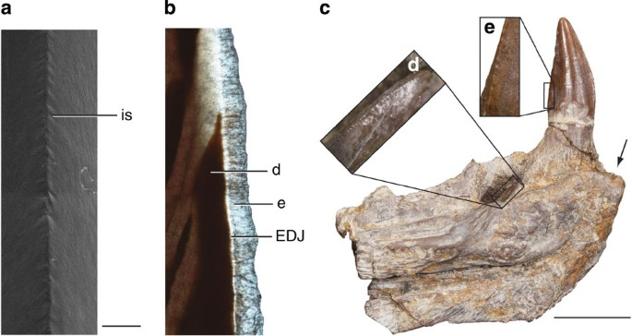Figure 3: cf.D. limbatusteeth. (a) Scanning electron microscope (SEM) of the distal carina of CMN (Canadian Museum of Nature) 9836 showing ornamentation of the enamel. (b) Thin section of Royal Ontario Museum 64021 mesial carina viewed under plain polarized light. (c) cf.D. limbatusSteinman Institute Division of Paleontology, University of Bonn 598 dentary teeth. Enamel ornamentation on distal carina of unerupted tooth (d) and erupted second dentary tooth (e). Black arrow indicates position of first dentary tooth. d, dentine; e, enamel; EDJ, enamel–dentine junction; is, interdentinal sulcus. Scale bars, (a) and (b), 0.5 mm, (c) 1 cm. Figure 3: cf. D. limbatus teeth. ( a ) Scanning electron microscope (SEM) of the distal carina of CMN (Canadian Museum of Nature) 9836 showing ornamentation of the enamel. ( b ) Thin section of Royal Ontario Museum 64021 mesial carina viewed under plain polarized light. ( c ) cf. D. limbatus Steinman Institute Division of Paleontology, University of Bonn 598 dentary teeth. Enamel ornamentation on distal carina of unerupted tooth ( d ) and erupted second dentary tooth ( e ). Black arrow indicates position of first dentary tooth. d, dentine; e, enamel; EDJ, enamel–dentine junction; is, interdentinal sulcus. Scale bars, ( a ) and ( b ), 0.5 mm, ( c ) 1 cm. Full size image The teeth from the Craddock Bonebed, cf. D. grandis (ROM 1797, ROM 6039, UMMP 55038), are ziphodont with large, well-defined denticles ( Fig. 4 ). All teeth examined have denticulate posterior carinae, but some teeth lack denticles on the mesial carinae. Not all denticles are equal in size; some are much larger apico-basally than others along the carina of the same tooth ( Fig. 4a,b ). The keel of each denticle is typically in-line with the keels of neighbouring denticles ( Fig. 4c ). When examined histologically, each denticle has a dentine core ( Fig. 4d,e ). Some specimens show cracks in the enamel between denticles ( Fig. 4e ), which could be interpreted as a ‘kerf and drill’ structure, similar to theropod dinosaurs [12] , although the base of the crack lacks an ampulla. It is difficult to determine whether the cracks were created in vivo or taphonomically, especially as the crack is not present between each denticle in every specimen. The morphology of the denticles differs between mesial and distal carinae. The mesial denticles are apically directed and asymmetrical, whereas the distal denticles are more symmetrical and have larger interdenticular distances ( Fig. 4d,e ). The dentine tubules are curved around the interdentinal space, following the EDJ ( Fig. 3d,e ). The thickness of the enamel varies along the carina, measuring 60 μm at the keel and 40 μm towards the interdentinal sulcus in both the mesial and distal carinae. Teeth from both small (presumed juveniles, for example, FMNH UC (Field Museum of Natural History) 1563) and large skulls (presumed adults, for example, FMNH UC 1636) have completely developed denticles. 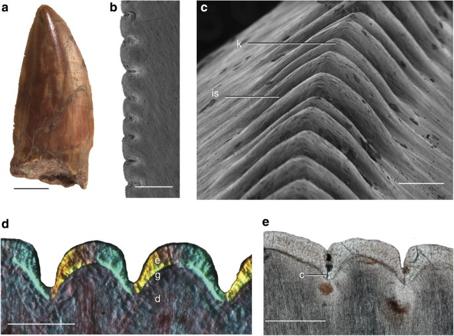Figure 4: cf.D. grandisteeth. (a) Royal Ontario Museum (ROM) 1797 tooth, labial view, mesial carina to the right. (b) ROM 1797, scanning electron microscope (SEM) of posterior carina, apical up. (c) ROM 6039, SEM of posterior carina, basal up. (d) ROM 6039Z, posterior carina, apical left. Viewed under cross-polarized light with a lambda plate and oblique illumination. (e) ROM 6039K, anterior carina, apical left. Viewed under plain polarized light. c, crack; d, dentine; e, enamel; g, globular dentine; is, interdentinal sulcus; k, keel. Scale bars, (a) 0.5 cm, (b–e) 0.5 mm. Figure 4: cf. D. grandis teeth. ( a ) Royal Ontario Museum (ROM) 1797 tooth, labial view, mesial carina to the right. ( b ) ROM 1797, scanning electron microscope (SEM) of posterior carina, apical up. ( c ) ROM 6039, SEM of posterior carina, basal up. ( d ) ROM 6039Z, posterior carina, apical left. Viewed under cross-polarized light with a lambda plate and oblique illumination. ( e ) ROM 6039K, anterior carina, apical left. Viewed under plain polarized light. c, crack; d, dentine; e, enamel; g, globular dentine; is, interdentinal sulcus; k, keel. Scale bars, ( a ) 0.5 cm, ( b – e ) 0.5 mm. Full size image The teeth of Secodontosaurus, Sphenacodon and Ctenospondylus are all similar to those of Dimetrodon in being recurved and labially convex ( Fig. 5 ). The teeth of Secodontosaurus do not possess dentine-cored serrations. The enamel is thick, resulting in a thickened carina on the tooth with many serrations, approximately nine to ten per mm. In erupted teeth, the longitudinal enamel ornamentation appears to converge towards the tip of the tooth ( Fig. 5a,b ). The enamel on the teeth is highly rugose, particularly in unerupted teeth ( Fig. 5c,d ). The enamel is 380 μm thick at the keel, and 150–250 μm thick along the mesial and distal carinae ( Fig. 5d ). On some teeth, the mesial carina curves lingually as in D. milleri and D. limbatus , but does not possess cusps. The teeth of Sphenacodon (for example, UCMP 34226, UMMP 9778, YPM (Yale Peabody Museum) 806, ROM 66534) and Ctenospondylus [30] have carinae with smooth cutting edges ( Fig. 5e,f ). None of the teeth examined displayed any serrated carinae, and most closely resemble the carinae of D. milleri, except there are no cusps on the lingual side of the teeth. Some teeth possess longitudinal fluting on the enlarged anterior cheek teeth of the maxilla and dentary ( Fig. 5f ). 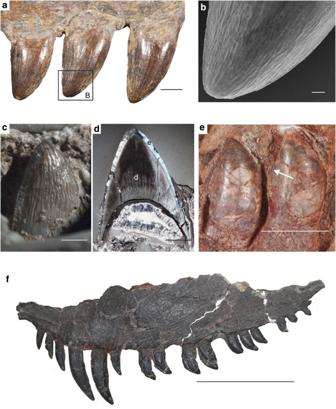Figure 5: Teeth of three sphenacodontids. (a) University of Michigan Museum of Paleontology 9714, maxillary teeth ofSecodontosaurus obtusidensin labial view, mesial right. (b) Scanning electron microscope (SEM) detail of (a) of the enamel near the tooth tip. (c) Erupting tooth ofS. obtusidens, Royal Ontario Museum (ROM) 6027, mesial to the right. (d) ROM 6027-AA1 thin section of (c) viewed in cross-polarized light, mesial right. (e)Sphenacodon ferocior, ROM 66534, dentary teeth in labial view. Arrow indicates tooth carina. (f) Museum of Comparative Zoology 3386, maxilla ofCtenospondylus ninevehensis, anterior left. The cutting edges ofC. ninevehensisare similar to those ofS. ferocior. d, dentine; e, enamel. Scale bars, (a) 2 mm, (b) 0.5 mm, (c) and (d) 1.5 mm, (e) 0.5 cm, (f) 5 cm. Figure 5: Teeth of three sphenacodontids. ( a ) University of Michigan Museum of Paleontology 9714, maxillary teeth of Secodontosaurus obtusidens in labial view, mesial right. ( b ) Scanning electron microscope (SEM) detail of ( a ) of the enamel near the tooth tip. ( c ) Erupting tooth of S. obtusidens , Royal Ontario Museum (ROM) 6027, mesial to the right. ( d ) ROM 6027-AA1 thin section of ( c ) viewed in cross-polarized light, mesial right. ( e ) Sphenacodon ferocior , ROM 66534, dentary teeth in labial view. Arrow indicates tooth carina. ( f ) Museum of Comparative Zoology 3386, maxilla of Ctenospondylus ninevehensis , anterior left. The cutting edges of C. ninevehensis are similar to those of S. ferocior . d, dentine; e, enamel. Scale bars, ( a ) 2 mm, ( b ) 0.5 mm, ( c ) and ( d ) 1.5 mm, ( e ) 0.5 cm, ( f ) 5 cm. Full size image Phylogenetic analysis of Sphenacodontoidea Tooth characters were examined in a phylogenetic analysis of Sphenacodontoidea using the character matrix of Fröbisch et al. [31] The resulting topology ( Fig. 6 ) is similar to that of Fröbisch et al. [31] Of the 122 characters, 72 are parsimony informative for Sphenacodontoidea. The three species of Dimetrodon are united by one unambiguous character (122): level of jaw articulation set below dentary tooth row. The topology of the tree did not change when character 51 was deleted from the analysis. By tracing the evolution of character 51 on the phylogeny, a complex pattern of tooth development emerges, where the development of ziphodonty is convergent between therapsids and some species of Dimetrodon , and enamel ornamentations are convergent between Secodontosaurus and species of Dimetrodon. The likelihood analysis suggests that there is a higher likelihood of enamel ornamentations evolving at each node rather than ziphodonty. The likelihood of enamel ornamentations evolving at node eight is due to the shortened amount of time between the node and the appearance of cf. D. limbatus ( Fig. 6 ). 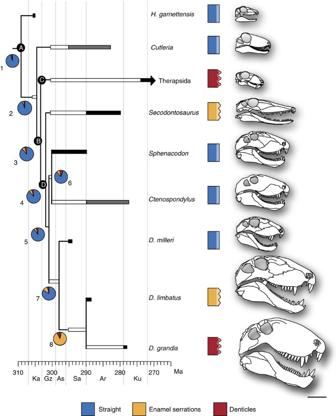Figure 6: Phylogeny of Sphenacodontoidea. Black indicates fossil occurrence, white indicates ghost lineages and grey indicates approximate age range. Pie charts indicate the likelihood of each character state evolving at that particular node. Blue represents teeth with straight-edged carinae, yellow represents teeth with crenulated enamel on the carinae, and red represents teeth with true denticles. Skull outlines are scaled to the largest known skulls of each species, as described in Romer and Price1. All skull outlines were adapted and redrawn from Reisz2, with the exception ofCutleriaandCtenospondylus. Tree statistics: length: 145; Consistency Index (CI): 0.9172; Retention Index (RI): 0.8723; Rescaled Consistency Index (RC): 0.8; Homoplasy Index (HI): 0.1132. A, Sphenacodontia; B, Sphenacodontoidea; C, Therapsida; D, Sphenacodontidae. Ar, Artinskian; As, Asselian; Gz, Gzhelian; Ka, Kasimovian; Ku, Kungurian; Ma, million years; Sa, Sakmarian. Scale bar, 10 cm. Figure 6: Phylogeny of Sphenacodontoidea. Black indicates fossil occurrence, white indicates ghost lineages and grey indicates approximate age range. Pie charts indicate the likelihood of each character state evolving at that particular node. Blue represents teeth with straight-edged carinae, yellow represents teeth with crenulated enamel on the carinae, and red represents teeth with true denticles. Skull outlines are scaled to the largest known skulls of each species, as described in Romer and Price [1] . All skull outlines were adapted and redrawn from Reisz [2] , with the exception of Cutleria and Ctenospondylus . Tree statistics: length: 145; Consistency Index (CI): 0.9172; Retention Index (RI): 0.8723; Rescaled Consistency Index (RC): 0.8; Homoplasy Index (HI): 0.1132. A, Sphenacodontia; B, Sphenacodontoidea; C, Therapsida; D, Sphenacodontidae. Ar, Artinskian; As, Asselian; Gz, Gzhelian; Ka, Kasimovian; Ku, Kungurian; Ma, million years; Sa, Sakmarian. Scale bar, 10 cm. Full size image This analysis of dental evolution in the oldest known terrestrial apex predators, the sphenacodontid synapsids, reveals three significant and unexpected result. First, the first occurrence of cusps in the evolutionary history of synapsid teeth is homoplastic with respect to the cusps of derived therapsids and mammals, and the cusps appear in sphenacodontids before the appearance of ziphodont teeth in Dimetrodon and therapsids. Second, ziphodonty is not present in all species of Dimetrodon , indicating that this important evolutionary novelty evolved within the genus. Last, there is previously undocumented diversity in tooth structure not only in Dimetrodon but also in other sphenacodontids, even though skull morphology is constrained in the clade. The presence and structure of the serrations and enamel ornamentation on the tooth carinae are therefore potentially useful for distinguishing between species of Dimetrodon and other sphenacodontids, whereas cranial anatomy typically does not [2] . The variation in dental anatomy within the broad designation of apex predatory dentition suggests that some interesting experimentation with tooth structure occurred at this early stage of terrestrial vertebrate evolution, before the appearance of a variety of cusped teeth in carnivorous therapsids, such as dinocephalians [32] and cynodonts [33] . An examination of skull morphology suggests that the shape and overall structure of the skull of sphenacodontids did not vary significantly between species ( Fig. 6 ), with the exception of the elongate skull of Secodontosaurus . The gross morphology of the teeth also did not vary significantly, as most sphenacodontids are heterodont with enlarged teeth at the front of the snout for holding prey, and smaller, recurved cheek teeth for piercing and slicing flesh. It is the microanatomy of the cheek teeth that show the most variation between taxa through time. Secodontosaurus has a temporal range of approximately 12 million years (Sakmarian–Kungurian), and co-occurs with Dimetrodon at both the Briar Creek and Craddock Bonebed localities. The morphology of the teeth in Secodontosaurus is similar at both localities in having elaborate apico-basal enamel ridges. This feature does not change throughout their evolutionary history, whereas the morphology of the teeth in Dimetrodon at both localities is different, as the earlier teeth have enamel ornamentations only, and the later teeth are ziphodont. Sphenacodon is also preserved at several localities that span a duration of approximately 10 million years (Gzhelian–Sakmarian) and overlap with Dimetrodon at certain localities in New Mexico, Utah, Colorado and Arizona [34] , [35] . Yet, similar to Secodontosaurus , the teeth of Sphenacodon do not change in morphology through time, in strong contrast to those of Dimetrodon . These results suggest that skull shape was generally conserved throughout the evolutionary history of Dimetrodon , but evolutionary changes in tooth structure and function were more diverse in the lineage. The differences in tooth morphology of Dimetrodon allow us to propose a hypothesis of evolutionary change in the development of tooth anatomy through time. In the earliest occurring species, D. milleri and D. limbatus , and in Secodontosaurus , the EDJ is smooth, and the shape of the carina was probably created through amelogenesis (the formation of enamel). Any features of the enamel, including interdentinal sulci, bumps and ridges, are composed of enamel only [36] . Enamel surface morphology is usually controlled by epithelial folding or differences in the timing of amelogenesis, where different crystals grow at different rates [28] , [29] , [37] . In later occurring species, such as D. grandis , the shape of the tooth was created by dentine, before the deposition of enamel. In these teeth, the EDJ is wavy along the carinae, creating the serrations. There is an upper limit to the size of enamel prisms that can be deposited on teeth, and so to develop large structures such as denticles, the shape must be pre-formed by the dentine before enamel deposition [36] . The initiation of shape in the dentine was most likely caused by the formation of enamel knots in tooth development [38] . The enamel of unerupted teeth examined here is thicker and more ornamented than the enamel of erupted teeth, in both Dimetrodon and Secodontosaurus ( Figs 3c–e and 4c,d ). These differences could be due to wear. However, the effect of ontogeny and tooth eruption on the morphology of the enamel is not known in any extinct taxon, and more developmental studies of enamel in reptiles are needed [37] , [39] . These results do raise the possibility that the pattern of enamel ornamentation on a tooth may vary ontogenetically. The presence of denticles on teeth from small, presumably juvenile skulls from the Craddock Bonebed (FMNH UC 1563) indicates that the development and maintenance of denticles on teeth at the same tooth position is more constrained and does not vary as much as the enamel ornamentation varies in other species through ontogeny. The role of gene expression in the development of carinae is unknown, as studies on tooth development in species of Varanus with denticulate carinae have never been performed [40] , [41] . The development of denticulate teeth in sharks is better known; however, they do not work well as a model for tooth development in amniotes as the pattern of denticles is not consistent between successive teeth in a single tooth family [42] , and the tooth tissues differ [43] , [44] . The shape of a tooth appears to correlate with the ecology of an animal, more specifically, its feeding behaviour [21] , [29] , [41] , [45] , [46] , [47] . Therefore, the evolution of ziphodonty within one clade of sphenacodontids suggests that feeding behaviour within the family may have changed over time, and different species of Dimetrodon dealt with their prey differently. Extensive modeling, morphometrics and proof of concept experiments have shown that ziphodont teeth are efficient at slicing and cutting prey items [11] , [12] , [16] , [19] , [20] , [48] . Abler’s [9] results suggest that serrations are more effective at puncturing and gripping food than teeth without serrations. The curvature of teeth suggests that they could bite and pull, but were most likely not used to crack bone [20] . Ziphodonty would therefore reduce the energy required to slice through prey items, allowing for more efficient feeding and enabling the animal to feed on large prey items, potentially prey items larger than itself [23] , [49] , and a stronger bite force [11] , [18] , [50] . Therefore, a change in tooth structure without a change in skull shape may have improved the feeding strategy of Dimetrodon over its 25 million year duration. The first occurrence of ziphodonty in Dimetrodon appears to correlate with faunal changes and body size changes in large-bodied Early Permian herbivores. The caseids become abundant in the Kungurian as diadectids and edaphosaurids decline in diversity [51] , [52] , and also increase in body size to be larger than their predatory coevals [1] . It remains to be quantitatively tested whether there is a correlation between changes in tooth structure and body size in Dimetrodon, and whether there are changes in body size between Dimetrodon and potential prey species. It is also possible that changes in tooth morphology in Dimetrodon may have been driven by competition between co-occurring sphenacodontid species. Description of sphenacodontid teeth Many shed and articulated teeth were examined macroscopically for this study from a variety of taxa, including Cutleria , Haptodus garnettensis , Dimetrodon , Secodontosaurus , Sphenacodon, Ctenospondylus and Alrausuchus . Materials of Dimetrodon , Secodontosaurus and Sphenacodon were collected from several Early Permian (Asselian–Kungurian) localities in Texas and New Mexico ( Supplementary Table 1 ). Some of these localities in Texas have produced co-occurring specimens of Secodontosaurus and multiple species of Dimetrodon : from the Archer City Bonebed: D. milleri ; from Mount Barry: D. natalis , D. limbatus and S. obtusidens ; from Briar Creek: D. natalis , D. booneorum , D. limbatus and S. obtusidens ; from Rattlesnake Canyon: D. natalis , D. booneorum and D. limbatus ; and from the Craddock bonebed: D. grandis, D. loomisi , D. giganhomogenes and S. obtusidens [1] , [53] , [54] . The majority of these taxa are differentiated from each other based on the size and proportions of postcranial elements [1] . Therefore, the taxonomic assignments of the disarticulated specimens used in this study are based on holotype material and the best known associated specimens from the localities of interest, as further detailed work on the taxonomy of Dimetrodon is required. Histological analysis of sphenacodontid teeth The marginal teeth of cf. D. limbatus (ROM 64021), cf. D. grandis (ROM 1797, ROM 6039) and S. obtusidens (ROM 6027) were analysed histologically for this study. Thin sections were made longitudinally through the carinae to examine the internal structure of the teeth, following the methodology of previous studies of tooth microstructure [28] , [55] , [56] , [57] , with some modification. Specimens were embedded in Castolite AP polyester resin and cut using a Buehler Isomet 1,000 wafer blade low-speed saw. Cut specimens were mounted to glass and plexiglass slides using Scotch-Weld SF-100 cyanoacrylate. Specimens were ground down to approximately 180 μm thick using a Hillquist grinding cup (Hillquist), then ground by hand using progressively finer grits of silicon carbide powder. Specimens were photographed using a Nikon DS-Fi1 camera mounted to a Nikon AZ-100 microscope (Nikon) fitted with crossed-polarizing and lambda filtres, and an oblique illumination slider. Thin section images were processed using Nikon NIS-Elements (Basic Research) v. 3.13 imaging software (Nikon). Specimens were also examined in a Jeol Neoscope JCM-5000 SEM (Jeol), which does not require sputter coating. Non-histological photographs were taken with a Canon Rebel T3i camera (Canon). Phylogenetic analysis of Sphenacodontoidea To examine the effect of tooth structure on the relationships of sphenacodontids, a phylogenetic analysis was performed using the character matrix of Fröbisch et al. [31] ( Supplementary Data 1 and Supplementary Methods ). The analysis was modified from Fröbisch et al. [31] to include only Sphenacodontoidea ( Dimetrodon , Secodontosaurus , Sphenacodon) , and Therapsida (represented by the taxon Alrausuchus ) in the ingroup, and Cutleria and Haptodus garnettensis in the outgroup, as these are the taxa with the most information on tooth morphology available for this study. The genus was split into three separate Operational Taxon Units (OTUs): cf. D. milleri, representing the Sakmarian Archer City Bonebed; cf. D. limbatus, representing the Artinskian Briar Creek and Rattlesnake Canyon localities; and cf. D. grandis, representing the Kungurian Craddock locality. A new character state was added to character 51 to code the differences in enamel and dentine serrations among taxa: marginal tooth serrations: absent (0); enamel only (1); dentine-cored (ziphodont) (2). The phylogeny was generated in Phylogenetic Analysis Using Parsimony (PAUP) using the branch-and-bound parsimony method [58] . Characters were unordered and unweighted. The resulting phylogeny was time calibrated using data from the literature [3] , [59] , [60] and the current geologic time scale [61] ( Supplementary Table 2 ). The scaled likelihoods of each ancestral state of the new character (51) at each node were calculated using an equal rates model in the package APE in R [62] ( Supplementary Table 3 ). Terminology used to describe sphenacodontid teeth In this study, ‘serrations’ refers to any bumps along the carina of a tooth, whether composed of enamel or by both dentine and enamel. We consider ziphodont teeth to possess ‘true’ denticles, which are serrations with dentine cores and enamel caps. The presence of ‘true’ denticles can only be accurately determined using histological methods. The occurrence of ziphodonty has been studied in depth in thalattosuchian crocodilians [15] , [18] , [23] , where different terminology was developed to denote true ziphodonty from ‘false ziphodonty’, which are enamel keels that appear similar to denticles through macroscopic examination. However, these terms describe specimens that were only examined using SEM, and the internal anatomy of the carinae is not known. Therefore, we prefer to distinguish between ziphodont teeth and teeth with enamel ornamentation on the basis of histological examination. How to cite this article: Brink, K. S. and Reisz, R. R. Hidden dental diversity in the oldest terrestrial apex predator Dimetrodon . Nat. Commun. 5:3269 doi: 10.1038/ncomms4269 (2014).